Organocatalytic enantioselective β-functionalization of aldehydes by oxidation of enamines and their application in cascade reactions Iminium catalysis, involving the transformation of iminium ions to enamines, has been extensively studied in the context of a number of organic processes. However, the reverse of this process involving conversion of enamines to iminium species has not been realized. Here, we describe a new transformation—'oxidative enamine catalysis'—in which direct oxidation of an enamine occurs to generate an iminium species. We show that the use of o -iodoxybenzoic acid as an oxidant in the presence of a secondary amine catalyst serves as effective system for promoting rapid conversion of enamines to iminium ions. The preparative power of this process has been demonstrated in the context of direct asymmetric β-functionalization of simple aldehydes. Moreover, a variety of enantioselective cascade transformations, including triple and quadruple cascades, have been developed for the 'one-pot' synthesis of versatile chiral building blocks and structural frameworks starting with simple aldehydes. Seminal independent investigations of enamine and iminium catalysis by List and Barbas [1] , [2] , [3] , [4] and MacMillan [5] , [6] , [7] serve as the conceptual basis for the field of organocatalysis. The field has grown at an explosive pace over the past decade and a number of unprecedented organic reactions have been discovered [3] , [4] , [6] , [7] , [8] . The success of aminocatalysis can perhaps be attributed to the unique activation modes that operate and the notable characteristics of their mechanistic features. In enamine catalysis ( Fig. 1a ), the formed reactive enamine contains an energetically elevated highest occupied molecular orbital (HOMO) in contrast to its aldehyde enol precursor. This leads to high reactivity with a wide range of electrophiles and subsequent generation of enantioenriched α-substituted products that arise by hydrolysis of the resulting iminium ions. In contrast, in iminium catalysis, the electrophilicity of α,β-unsaturated carbonyls such as enals is enhanced by formation of corresponding iminium ions that possess low lowest unoccupied molecular orbital (LUMO) energies ( Fig. 1b ). As a consequence, the intermediates α,β-unsaturated iminium species react with a diverse array of nucleophiles giving adducts that are obtained through subsequent hydrolysis of corresponding enamines. It is recognized that in these catalytic processes, enamine and iminium intermediates exist in rapid equilibrium. Recently, MacMillan introduced a third type of catalysis involving singly occupied molecular orbital (SOMO) activation mode for α-functionalization of aldehydes ( Fig. 1c ) [9] , [10] . Remarkably, the three generic activation modes presented above have been used in a large number of unprecedented enantioselective organic transformations [11] , which are complementary to those promoted by organometallic catalysts. Furthermore, capitalizing on reversible iminium-enamine catalysis ( Fig. 1b ), a number of synthetically efficient catalytic enantioselective cascade processes have been developed for the facile construction of complex molecular architectures [12] , [13] , [14] . 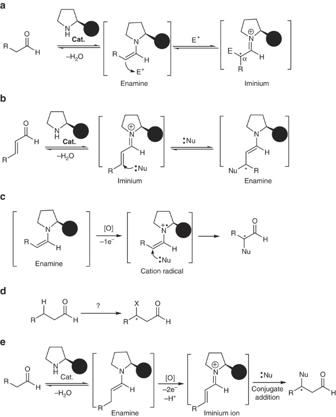Figure 1: Aminocatalysis. (a) Enamine catalysis. (b) Iminium catalysis. (c) SOMO catalysis. (d) Direction catalytic enantioselective β-functionalization of aldehydes remains elusive. (e) Proposed oxidative enamine catalysis: 'one-pot' access to β-functionalization aldehydes from simple aldehydes. Figure 1: Aminocatalysis. ( a ) Enamine catalysis. ( b ) Iminium catalysis. ( c ) SOMO catalysis. ( d ) Direction catalytic enantioselective β-functionalization of aldehydes remains elusive. ( e ) Proposed oxidative enamine catalysis: 'one-pot' access to β-functionalization aldehydes from simple aldehydes. Full size image Although enamine and SOMO catalysis represent powerful approaches to α-functionalization of aldehydes ( Fig. 1a,c ), to our knowledge, methods for direct β-functionalization of simple aldehydes rather than enals in a catalytic enantioselective manner have not been reported ( Fig. 1d ). With the aim of expanding the scope of aminocatalysis beyond the three activation modes described above ( Fig. 1d ), we recently questioned whether it would be possible to devise a new aminocatalysis strategy. Although the strategy involving transformation of an iminium ion to an enamine in iminium catalysis has enjoyed tremendous successes ( Fig. 1b ), the reverse process in which an enamine is converted to an iminium species has not been explored. Given the established capacity of iminium and enamines species to interconvert by a redox process, we believed that it might be feasible to transform an enamine into an iminium ion ( Fig. 1e ). Specifically, we hypothesized that oxidation of electron-rich enamine derived from an aldehyde and a chiral amine would give rise to an iminium ion through a process termed 'oxidative enamine catalysis'. The resulting iminium species would then undergo enantioselective conjugation addition (functionalization) to form a new chiral C–Nu bonded product. Although the proposed catalytic conversion of an enamine to an iminium species at first sight appears simple, its realization is faced with several challenging issues. At the outset, we understood that the widespread application of oxidative enamine catalysis would require the identification of an oxidant that would selectively oxidize the enamine through a 2e − transfer pathway to generate a requisite α,β-unsaturated aldehyde-derived iminium ion. Second, the amine catalyst would need to be inert under the oxidation reaction conditions, a potentially difficult task, as studies have shown that secondary amines are readily oxidized to form imines [15] . Third and important, the intrinsic value of this new process would be defined by its capacity to enable useful enantioselective transformations. Moreover, owing to the sensitive dependence of reaction yields and levels of enantio- and/or diastereoselectivity to reaction conditions, the oxidant and resulting byproduct(s) should not interfere with or at least have minimal effects on the subsequent asymmetric conjugate addition process (for example, functionalization). Finally, the reaction medium should be compatible with both the oxidation and conjugate addition reactions to enable the achievement of high reaction efficiencies. The novel oxidative enamine catalysis strategy has potential because the enal-derived iminium ions are already known to participate in many C–C, C–O and C–N bond-forming processes. Therefore, a wide range of synthetically efficient, catalytic enantioselective transformations should occur in a cascade manner. In this study, we find that the use of o -iodoxybenzoic acid (IBX) as an oxidant in the presence of a secondary amine catalyst serves as an effective system for promoting rapid conversion of enamines to iminium ions. The process is demonstrated in the context of direct asymmetric β-functionalization of simple aldehydes. Furthermore, a variety of novel enantioselective cascade transformations, including triple and quadruple cascades, have been developed for the 'one-pot' synthesis of versatile chiral building blocks and structural frameworks. The operational simplicity and mild reaction conditions involved in these processes make them particularly attractive. Exploration studies Recently, we described an amine-Pd(OAc) 2 co-catalysed Saegusa-type reaction involving the transformation of aldehydes to enals ( Supplementary Fig. S1 ) (ref. 16 ). Mechanistically, the reaction involves Pd(OAc) 2 catalysed oxidation of an enamine, serving as an equivalent of silyl enol ether in a typical Saegusa reaction, in the presence of O 2 to produce a corresponding conjugated iminium ion. Unfortunately, the relatively restricted reaction conditions (DMSO as an essential solvent, and elevated reaction temperatures) that are required to make the process inapplicable to subsequent asymmetric conjugate addition reactions. However, the important insight gained from studies of this process is that direct oxidation of an enamine to a conjugated iminium ion is possible. This observation provided a foundation for us to explore oxidative enamine catalysis of direct enantioselective β-functionalizations of aldehydes. To demonstrate the feasibility of the proposed oxidation-conjugate addition reaction, fluorobis(phenylsulfonyl)methane (FBSM, 2 ) [17] was selected as the nucleophile for the subsequent Michael addition process, as the FBSM moiety can be conveniently converted to the synthetically and medicinally significant monofluoromethyl group. As a result, the process would serve as a valuable method for asymmetric synthesis of chiral fluorinated compounds [18] . A model reaction between 3-phenylpropionaldehyde ( 1a , R=Ph) and FBSM was carried out in the presence of diphenylprolinol trimethylsilyl (TMS) ether ( I ) ( Table 1 ) [19] , [20] , [21] , a widely used organocatalyst in aminocatalysis, in CH 2 Cl 2 at room temperature (RT; Table 1 , entry 1). Screening of several oxidants (entries 1–6) showed that the use of IBX was encouraging. In this case, the desired product 3a was obtained albeit low yield (10%) and with only a moderate degree of enantioselectivity (71% ee). In contrast, other oxidants including CAN, a reagent used in MacMillan's SOMO catalysis [9] , failed to promote formation of 3a (entries 2–6). Moreover, when IBX was used for the oxidation process under the conditions reported by Nicolaou et al . [22] , [23] (entries 6 and 8), a complicated mixture of products was obtained that did not contain the desired product. Table 1 Exploration of amine catalyzed enantioselective direct β-functionalization of 3-phenyl-propionaldehyde*. Full size table IBX was chosen as the oxidant for further optimization of the conditions for the oxidation-conjugate addition reaction. We thought that the low yield observed initially might be a consequence of the poor solubility of IBX in CH 2 Cl 2 . Accordingly, a commonly used solvent for IBX-mediated oxidation reaction, DMSO, was used ( Table 1 , entry 7), but surprisingly no reaction took place. However, the use of ethanol as solvent for the IBX-mediated process lead to a considerably improved yield (entry 9, 55%), but a lower ee (55%) was observed. Among the solvents probed, it appeared that toluene was optimal for the cascade process (entry 11). Using this solvent, a 24% yield and 76% ee were obtained for the IBX promoted reaction of 1a with FBSM. Lowering the reaction temperature to 0 °C and prolonging the reaction time led to a significant enhancement in both yield and percentage of ee (entry 12, 56% yield and 92% ee). Screening analogues II – IV of catalyst I revealed that although enantioselectivities were improved (entries 14 and 15) the yields were lowered and IV did not promote the process at all (entry 16). Increasing catalyst loading (30 mol%, entry 13) led to an improvement in the reaction yield (62%) without affecting the level of enantioselectivity. It should be noted that the chiral amine catalyst used in this process can be oxidized to an imine by IBX [15] . This is the major reason why a high catalyst loading is required. Scope of organocatalytic enantioselective β-functionalizations The established optimal reaction conditions were used in an exploration of the scope of the β-functionalization process with FBSM ( 2 ) as the nucleophile. The results show that I catalysed asymmetric cascade IBX–oxidation–Michael reactions of aldehydes with FBSM proceed with high enantioselectivity and in good yields, and with a broad substrate range ( Fig. 2 ). Both aromatic and aliphatic aldehydes effectively participate in the cascade process. It is noteworthy that the efficiency of the cascade process is comparable to that of single Michael additions of FBSM to enals catalysed by the TBDMS analog of I , a process recently developed by us and Moyano and Rios [24] , [25] . 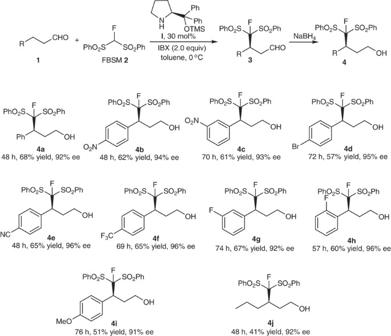Figure 2: Organocatalytic enantioselective cascade oxidation-Michael reactions with FBSM. Unless stated otherwise, seeMethodsfor details of the reaction conditions. OTMS, trimethlsilyloxy. Figure 2: Organocatalytic enantioselective cascade oxidation-Michael reactions with FBSM. Unless stated otherwise, see Methods for details of the reaction conditions. OTMS, trimethlsilyloxy. Full size image To demonstrate the broad utility of this direct β-functionalization strategy, we probed reactions involving other carbon-centered nucleophiles such as malonates 5 ( Supplementary Fig. S2 ) (ref. 26 ). Studies showed that optimal reaction conditions involved the use of catalyst I , IBX and the essential additive NaOAc in toluene at RT (see Supplementary Information for details). High enantioselectivities (89–97% ee) were found to accompany the I -promoted cascade IBX–oxidation–Michael reaction of aldehydes with malonates. Oxidative enamine catalysis in cascade processes Preliminary results from investigations of a variety of multiple step (more than two steps) cascade reactions ( Fig. 3 ) serve as a testament to the versatility and power of oxidative enamine catalysis. For example, both aldehydes 1a and 7 undergo triple cascade oxidation–Michael–cyclization reactions with 4-hydroxycoumarin ( 8 ) to produce biologically interesting coumarin-containing chiral pyran 9 with useful levels of enatioselectivity and in good yields ( Fig. 3a ) (ref. 27 ). 1,3-Cyclohexandione ( 11 ) can be used as a nucleophile in the reaction of aldehyde 11 that leads to construction of the structurally diverse pyran 12 with high enantioselectivity (90% ee, Fig. 3b ). It should be noted that when 11 is added together with 10 , catalysts I and IBX, a lower reaction yield (45%) is obtained. In addition to carbon nucleophiles, O - and N -centered nucleophilic substances also participate in oxidative enamine cascade catalysed, quadruple cascade oxidation–Michael–aldol-dehydration processes ( Fig. 3c,d ) (refs 28 , 29 ). Although 4 Å molecular sieves (MS) are used in this process to facilitate dehydration, a certain amount of water is essential for the formation of products 14 and 16 . Furthermore, intramolecular versions of the oxidative enamine cascade catalysis have been devised, which afford synthetically and biologically useful, complex, chiral dihydro-isoindole 18 and spirooxindole 20 frameworks in 'one-pot' operations ( Fig. 3e,f ) (ref. 30 ). 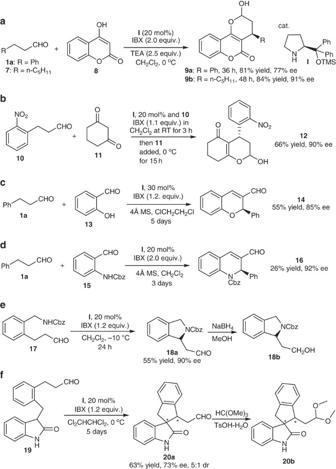Figure 3: Organocatalytic enantioselective triple and quadruple cascade reactions. (a,b) Triple cascade oxidation–Michael–cyclization reactions. (c,d) Oxidation–Michael–aldol-dehydration reactions. (e,f) Intramolecular oxidation-Michael reactions. SeeSupplementary Methodsfor detailed reaction conditions. TEA, triethanolamine. Figure 3: Organocatalytic enantioselective triple and quadruple cascade reactions. ( a , b ) Triple cascade oxidation–Michael–cyclization reactions. ( c , d ) Oxidation–Michael–aldol-dehydration reactions. ( e , f ) Intramolecular oxidation-Michael reactions. See Supplementary Methods for detailed reaction conditions. TEA, triethanolamine. Full size image The novel organocatalytic oxidative enamine methodology involves a key transformation in which an in situ formed enamine derived from a corresponding aldehyde is converted to an iminium ion. To verify that this reaction pathway is actually followed in the process, we have conducted a series of control experiments. As the oxidation reaction results in the formation of an α,β-unsaturated aldehyde-derived iminium species, one would expect that hydrolysis of this intermediate would produce an enal product. Thus, reaction of 3-phenylpropionaldehyde ( 1a ) with organocatalyst I (10 mol%) and IBX (1.5 equiv.) without a nucleophile present at RT in toluene ( Supplementary Table S1 , entry 1) was carried out under similar conditions used in the oxidation–Michael cascade process (see Fig. 2 ). This reaction generated trans -cinnamaldehyde ( 21a ) in 78% yield (entry 1). In addition, controls using the tertiary amine triethanolamine as a possible catalyst or the absence of I did not result in formation of the desired product 21a , indicating that formation of an enamine is essential for the process (entries 2 and 3). For comparison purposes, we also used the conditions reported by Nicolaou et al . [22] , [23] for the oxidation step. In these cases, the reactions were highly solvent dependent (entries 5–7) and, as Nicolaou et al . reported, only DMSO was effective for formation of 21a . Interestingly, with the Nicolaou protocol large excesses of IBX (2.4 equiv.) and NMO (2.4 equiv) are required along with much longer reaction times (28 h) and a lower yield (58%) is obtained (entry 7). In addition, this process is not clean, producing several unidentified byproducts. Although IBX has a high solubility in DMSO, the amine-catalysed oxidation reaction using this oxidant in DMSO (entry 4) takes place as efficiently as those in non-polar solvents such as toluene (entry 1) and CH 2 Cl 2 (entry 8). Two possible reaction pathways are plausible for the amine-catalysed IBX oxidation process. One involves single electron transfer (SET; Fig. 4a ), whereas the other is an ionic process involving an electron pair transfer ( Fig. 4b ). Nicolaou et al . [22] , [23] proposed that, in a manner similar to CAN-mediated oxidations of enamines [9] , a SET mechanism and cation radical intermediates are involved in IBX promoted oxidation reactions transforming ketones to enones [26] . However, we have found that enal 21a is formed using the typical SET oxidant ceric ammonium nitrate (CAN) in dimethoxy ethane (DME) in the presence of diphenylprolinol TMS ether I . This observation suggests that the SET mechanism might not be operable in the new oxidation process. Alternatively, an ionic mechanism involving 2e transfer is possible ( Fig. 4b ). The pathway, which involves formation of iodic ester and subsequent elimination [31] , [32] , is similar to that used to explain IBX-mediated oxidations of alcohols to carbonyl products. 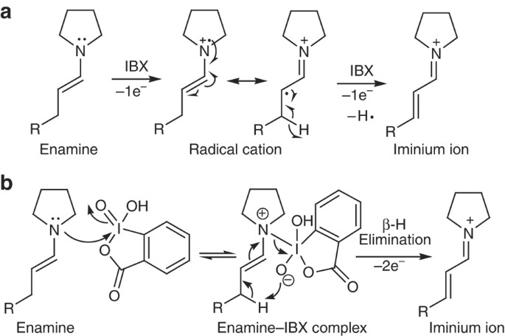Figure 4: Proposed mechanisms for amine-catalysed oxidation of enamines to iminium ions. (a) Single electron transfer (SET) pathway. (b) Ionic process involving an electron pair transfer. Figure 4: Proposed mechanisms for amine-catalysed oxidation of enamines to iminium ions. ( a ) Single electron transfer (SET) pathway. ( b ) Ionic process involving an electron pair transfer. Full size image In conclusion, this study has resulted in the development of an unprecedented organocatalytic method for enantioselective β-functionalization of simple aldehydes, involving oxidative conversion of enamines to iminium species and using a simple amine catalyst and the non-toxic IBX as oxidant. The methodology can also be viewed as an enantioselective C–H activation/functionalization process using an organocatalyst. Moreover, the synthetic potential of the oxidative enamine catalysis process was demonstrated by its application in a series of asymmetric cascade processes, including highly synthetic efficient triple and quadruple cascade sequences that result in 'one-pot' creation of complex molecular architectures. Mechanistic studies reveal that the process involves a transformation of an aldehyde to an enamine, which then undergoes oxidative conversion to an iminium ion. The novel transformation holds great potential for application to a broad spectrum of novel organic reactions that, along with the detailed mechanistic features of the oxidation process, serves to guide our further efforts in this area. General procedure for oxidation–Michael addition reactions General procedure for oxidation–Michael addition reactions. Aldehyde 1 (0.10 mmol), IBX (28 mg, 0.10 mmol), 2 (15.7 mg, 0.05 mmol) and catalyst I (4.9 mg, 0.015 mmol) were dissolved in toluene (0.6 ml) ( Fig. 2 ). The reaction mixture was stirred at 0 °C for the shown time, and then subjected to column chromatography (eluted with EtOAc/hexane) to afford aldehyde 3 . The resulting aldehyde 3 was dissolved in 1.0 ml of MeOH, then was cooled to 0 °C. NaBH 4 (11 mg, 0.3 mmol) was added in three portions and the resulting mixture was stirred at 0 °C for 20 min. The reaction mixture was poured into water and extracted with CH 2 Cl 2 (×3). The combined organic layers were washed with water and brine, dried (Na 2 SO 4 ) and concentrated. The residue was subjected to column chromatography (eluted with EtOAc/hexane) to afford alcohol 4 . Synthesis of compound 9a A mixture of dihydrocinnamaldehyde 1a (0.2 mmol, 2.0 equiv. ), IBX (0.2 mmol, 2.0 equiv.) and catalyst I (0.02 mmol, 20 mol%) in CH 2 Cl 2 (1 ml) was stirred at RT for 1 h. Then the mixture was cooled to 0 °C and Et 3 N (0.25 mmol, 2.5 equiv.) and 4-hydroxycoumarin 8 (0.1 mmol) were added. The mixture was stirred at the same temperature for 36 h and then subjected to column chromatography on silica gel to afford the desired product in 81% yield. Synthesis of compound 12 A mixture of 10 (0.1 mmol), IBX (0.11 mmol, 1.1 equiv.) and catalyst I (0.02 mmol, 20 mol%) in CH 2 Cl 2 (0.4 ml) was stirred at RT for 3 h. Then the mixture was cooled to 0 °C and then 11 (0.2 mmol) was added. The reaction was stirred at the same temperature for 15 h. The crude product was subjected to column chromatography on silica gel to afford the desired product in 66% yield. Synthesis of compound 14 A mixture of 1a (0.1 mmol), IBX (0.12 mmol, 1.2 equiv. ), compound 13 (1.0 mmol, 10 equiv.) and catalyst I (0.03 mmol, 30 mol%) in ClCH 2 CH 2 Cl (0.5 ml) were stirred at RT for 2 h. Then the mixture was cooled to 0 °C and 4 Å MS (50 mg) was added. The reaction was stirred at the same temperature for 5 days. The crude product was purified by column chromatography on silica gel to afford the desired product in 55% yield. Synthesis of compound 18 A mixture of 17 (0.20 mmol), IBX (0.24 mmol, 1.2 equiv.) and catalyst I (0.04 mmol, 20 mol%) in CH 2 Cl 2 (0.8 ml) was stirred at −10 °C for 24 h. The crude product was purified by column chromatography on silica gel to afford the desired product 18a in 55% yield. Aldehyde 18a was dissolved in MeOH (3.0 ml) then NaBH 4 (37.8 mg, 1.0 mmol) was added in three portions. The resulting mixture was stirred at RT for 20 min. The reaction mixture was poured into water and extracted with EtOAc for three times. The combined organic layers were then washed with water and brine, dried (Na 2 SO 4 ) and concentrated. The residue was then subjected to silica gel chromatography to give the corresponding alcohol 18b . Synthesis of compound 20 A mixture of 19 (0.10 mmol), IBX (0.12 mmol, 1.2 equiv.) and catalyst I (0.02 mmol, 20 mol %) in ClCH 2 CH 2 Cl (0.4 ml) was stirred at 0 °C for 5 days. The crude product was purified by column chromatography on silica gel to afford the desired product 20a in 63% yield. Aldehyde 20a was dissolved in MeOH (2.0 ml), HC(OMe) 3 (1.0 mmol) and TsOH·H 2 O (0.10 mmol) were added and the resulting mixture was stirred at RT for 1 h. The reaction mixture was poured into saturated aqueous NaHCO 3 and extracted with EtOAc for three times. The combined organic layers were then washed with water and brine, dried (Na 2 SO 4 ) and concentrated. The residue was then subjected to silica gel chromatography to give the corresponding alcohol 20b . How to cite this article: Zhang, S. et al . Organocatalytic enantioselective β-functionalization of aldehydes by oxidation of enamines and their application in cascade reactions. Nat. Commun. 2:211 doi: 10.1038/ncomms1214 (2011).